Release of SOS2 kinase from sequestration with GIGANTEA determines salt tolerance inArabidopsis Environmental challenges to plants typically entail retardation of vegetative growth and delay or cessation of flowering. Here we report a link between the flowering time regulator, GIGANTEA (GI), and adaptation to salt stress that is mechanistically based on GI degradation under saline conditions, thus retarding flowering. GI, a switch in photoperiodicity and circadian clock control, and the SNF1-related protein kinase SOS2 functionally interact. In the absence of stress, the GI:SOS2 complex prevents SOS2-based activation of SOS1, the major plant Na + /H + -antiporter mediating adaptation to salinity. GI overexpressing, rapidly flowering, plants show enhanced salt sensitivity, whereas gi mutants exhibit enhanced salt tolerance and delayed flowering. Salt-induced degradation of GI confers salt tolerance by the release of the SOS2 kinase. The GI–SOS2 interaction introduces a higher order regulatory circuit that can explain in molecular terms, the long observed connection between floral transition and adaptive environmental stress tolerance in Arabidopsis . Salt stress in plants includes an osmotic component that can lead to desiccation as the external osmotic potential declines with increasing salt concentrations, as well as a metabolic component as the influx of Na + disturbs signalling pathways, protein stability and biochemical reactions [1] . All plants can activate defense mechanisms whose complexity and amplitude depend on genetic complexity and allele structure and to some degree also on the memory of prior salt-stress episodes [2] . Although many salinity stress defense genes and pathways have been outlined [2] , [3] , the salt overly sensitive (SOS) pathway that appears to present a first line of defense has emerged as singularly important in studies using Arabidopsis thaliana . Salt stress can elicit growth reduction by ABA- and gibberellins (GA)-mediated (DELLA-dependent) signalling that extends the vegetative phase and inhibits flowering [4] , [5] , [6] , but the precise mechanism remains unknown. This growth restraint is active and distinct from salt-induced damage. To curtail salt-induced damage, salt-exposed plants maintain low cytosolic Na + concentrations by controlling influx, activating efflux, enhancing intracellular compartmentalization and coordinating tissue distribution of the ion. Efficient efflux of Na + is achieved in plants by the plant-specific SOS pathway, which re-establishes ion and, in part, water homeostasis after exposure to high salinity [7] , [8] . Among the three known proteins in this pathway, SOS1 is a Na + /H + antiporter regulated positively by a protein kinase complex comprised of the Ca 2+ activated protein SOS3 and the kinase SOS2, which phosphorylates SOS1 in response to salinity stress [7] , [9] . The transition from vegetative to reproductive growth is a key event in the life cycle of plants, constituting a crucial determinant of the reproductive success of the organism [10] . Timing of the floral transition is coordinated by a clock that controls the progression of development through genetic and epigenetic programming [11] , [12] , [13] . The floral transition requires triggering the initiation of flowering [14] , [15] , and also involves complex redeployment of a variety of metabolic and biochemical processes [16] , [17] . A plant’s environmental history and physiological status is connected to the timing of floral transition because it affects the prospects of survival and adaptation. Although the observational data are often anecdotal, cause and effect have occasionally become established and their genetic foundation corroborated [18] . Usually however, observations of correlations list participants, but fail to provide molecular genetics or biochemical insights into underlying mechanisms. Although mutations in genes first classified as regulating flowering time have been repeatedly observed to have pleiotropic effects on plant responses to environmentally activated signals, the biochemical processes involved in these interactions are poorly understood [4] , [19] , [20] , [21] . Here, we demonstrate that the flowering time gene GIGANTEA ( GI ) is a major component of the salt-stress adaptation pathway. Although other roles for GI have been reported [22] , it is predominantly associated with the promotion of flowering in long-day growth. GI is known to be a key component in the photoperiodic control pathway of flowering [23] , [24] , where it mediates light input to the circadian clock. Our results identify GI as the central module in a pathway that responds to the sensing of salinity stress conditions by delaying the initiation of flowering while providing stress tolerance. We report that GI is a strong negative regulator of salinity stress tolerance. GI cages SOS2 to the nucleoplasm and cytoplasm under normal growth conditions, but is degraded in response to salt stress. This then frees SOS2 to activate the plasma membrane-localized SOS1 Na + /H + -antiporter responsible for the export of sodium ions, which has so far been considered the key plant salt defense mechanism. These results provide a unique insight into a molecular mechanism that connects developmental stage transition and environmental stress tolerance in Arabidopsis . GI integrates salinity stress response and flowering time In Arabidopsis , flowering is induced by exposure to long days, with GI recognized as a key component in the photoperiodic control of flowering [23] , [24] , [25] , [26] . GI regulates the precise timing of expression of CONSTANS ( CO ), a transcriptional activator of the floral integrator gene Flowering Locus T ( FT ). To examine whether salinity stress provided a signal that affected the timing information in photoperiodic flowering, we first probed for the effects of elevated salinity on floral transition in gi mutants that lack GI functional protein. Under long-day conditions, WT phenocopies the gi mutant upon salt stress ( Fig. 1a and Supplementary Figs S1 and S2 ). All gi mutants flowered later than WT in the absence of NaCl. The flowering time of gi-1 , gi-2 and gi-201 was unaffected in media containing NaCl ( Fig. 1a and Supplementary Figs S1 and S2a,b ). CO and FT transcript levels were remarkably reduced by salt stress in WT, and their levels were low and not affected further by salt in gi-1 ( Fig. 1c ) providing an explanation for the abrogation of NaCl-induced delay of flowering in the gi-1 mutant. GI thus emerged as a player in orchestrating salt-induced late flowering in Arabidopsis . 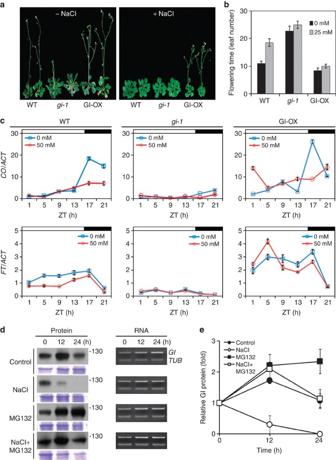Figure 1: GI regulates the initiation of flowering in response to salt stress. (a,b) Salt treatments delay flowering inArabidopsis. WT (Col-0),gi-1and GI-OX (35S::GI-HA) plants were grown under long-day conditions (16 h light/8 h dark) on MS media without and with 50 mM (a) or 25 mM NaCl (b) supplement. Plants were photographed at 5 weeks. Mean (±s.e.) flowering times are shown as number of leaves at bolting. (c) Effect of salt treatment on expression pattern of the flowering time regulator genesCOandFT. Twenty four hours NaCl treatment (0 and 50 mM) of 10-day-old seedlings grown on MS media was initiated at ZT0 (Zeitgeber time 0). Transcript levels, normalized to the transcript level ofActin(ACT), were measured by real-time qRT–PCR. Data are the mean±s.e. from three biological replicates. (d) GI is degraded upon exposure to salt in a proteasome-dependent manner. Detached leaves of soil-grown 3-week-old GI-OX plants were treated with NaCl (100 mM), MG132 (100 μM) or NaCl plus MG132 at ZT1. GI protein level (GI-HA, left panel) was evaluated after 0, 12 and 24 h treatments by immunoblot analysis with anti-HA antibody. Coomassie brilliant blue (CBB)-stained blots are shown as loading control. Molecular weight markers in kDa.GIandTubulin(TUB, internal control) transcript levels (right panel) were evaluated by RT–PCR. All experiments were repeated at least three times. (e) Quantification of the results shown in (d, left panel). Relative GI protein (fold) is the ratio of the GI signal at a given time to the GI signal at ZT0. Values represent mean±s.e. (n=3). Figure 1: GI regulates the initiation of flowering in response to salt stress. ( a , b ) Salt treatments delay flowering in Arabidopsis . WT (Col-0), gi-1 and GI-OX ( 35S::GI-HA ) plants were grown under long-day conditions (16 h light/8 h dark) on MS media without and with 50 mM ( a ) or 25 mM NaCl ( b ) supplement. Plants were photographed at 5 weeks. Mean (±s.e.) flowering times are shown as number of leaves at bolting. ( c ) Effect of salt treatment on expression pattern of the flowering time regulator genes CO and FT . Twenty four hours NaCl treatment (0 and 50 mM) of 10-day-old seedlings grown on MS media was initiated at ZT0 (Zeitgeber time 0). Transcript levels, normalized to the transcript level of Actin ( ACT ), were measured by real-time qRT–PCR. Data are the mean±s.e. from three biological replicates. ( d ) GI is degraded upon exposure to salt in a proteasome-dependent manner. Detached leaves of soil-grown 3-week-old GI-OX plants were treated with NaCl (100 mM), MG132 (100 μM) or NaCl plus MG132 at ZT1. GI protein level (GI-HA, left panel) was evaluated after 0, 12 and 24 h treatments by immunoblot analysis with anti-HA antibody. Coomassie brilliant blue (CBB)-stained blots are shown as loading control. Molecular weight markers in kDa. GI and Tubulin ( TUB , internal control) transcript levels (right panel) were evaluated by RT–PCR. All experiments were repeated at least three times. ( e ) Quantification of the results shown in ( d , left panel). Relative GI protein (fold) is the ratio of the GI signal at a given time to the GI signal at ZT0. Values represent mean±s.e. ( n =3). Full size image Salt-induced delay in flowering was completely suppressed in a GI-OX line that constitutively overexpresses GI . CO and FT are not reduced in a similar way as in WT, indicating that both the timing and expression level of GI are important for NaCl-induced delay of flowering ( Fig. 1a and Supplementary Fig. S1 ). GI expression is under control of the circadian clock [24] , [27] , [28] and the cellular level of GI protein is also subject to diurnal oscillation in part due to its dark-induced proteasomal degradation [29] . To evaluate the nature of the delay in flowering in response to salt treatment, GI protein and mRNA were therefore examined in plants expressing HA-tagged GI ( GI::GI-HA ) at close to WT levels. As shown by qRT–PCR, transcript levels of GI were enhanced upon salt treatment ( Supplementary Fig. S3c ). This might suggest that GI itself is gated by salt. To test for this possibility, the acute salt response of GI transcript levels was examined by 1 h salt treatments at different times of the day. We observed no significant response in GI transcript levels with 1 h salt treatments except for an increase at ZT8, the time point when GI transcript levels peak under control conditions ( Supplementary Fig. S3d ). This suggests that an effect of salt on GI transcripts is indirect. Although GI transcript level was enhanced, GI protein level was reduced in seedlings upon salt treatment although the diurnal cycling pattern was not affected ( Supplementary Fig. S3a–d ). For confirmation, GI protein and mRNA levels were examined in detached leaves of GI overexpressing plant ( 35S::GI-HA ). As in seedlings, the steady-state level of GI protein decreased and GI mRNA abundance increased upon salt treatment in a time-dependent manner ( Fig. 1d ). Inclusion of MG132, a proteasome inhibitor, during salt treatment abolished the NaCl-induced decrease in the steady-state levels of GI protein ( Fig. 1d ) indicating GI removal upon salt stress also depends on a functional proteasome complex. Regulated GI protein stability could be transmitted through the status of CO ( Fig. 1c ) thus causing salt-induced delay in flowering. These results explain why the NaCl-induced delay in flowering time depends on the expression of GI. Increased Na + /H + exchange activity in gi-1 plants We next examined whether GI might have a role in the regulation of salt stress responses by examining the salt-stress response of lines differing in GI activity. WT, gi-1 and GI-OX lines were grown in soil for2 weeks and then treated with 150 mM NaCl every 4 days for 2 weeks. In the absence of salt, soil-grown gi-1 plants showed improved vegetative and delayed reproductive growth in soil compared with WT ( Fig. 2a ). The gi-1 plants were more tolerant to NaCl than WT. Conversely, GI-overexpressing plants showed reduced vegetative but accelerated reproductive growth in the absence of salt, and were more sensitive to NaCl than WT. ( Fig. 2a ). These results suggest that GI functions as a negative factor interfering with mechanisms leading to salt tolerance. 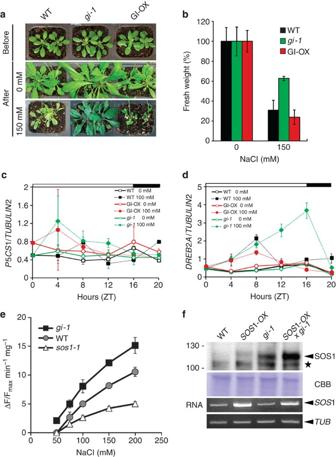Figure 2: Salt tolerance in thegimutant is mediated by increased Na+/H+exchange activity. (a,b) Thegimutant exhibits increased salt tolerance. (a) WT,gi-1and GI-OX plants were grown on soil for 3 weeks (top panel) and then treated with 0 mM (middle) or 150 mM (bottom) NaCl for 2 weeks. Plants are shown (a) representative of 10 to 12 individual plants that were examined for each line. (b) Fresh weight at the end of the treatments shown in (a). Index indicates the per cent decrease in average fresh weight after NaCl treatment. Data represent the mean±s.e. of the three independent replicates. (c,d) qRT–PCR analysis ofP5CS1(c) andDREB2A(d) transcript levels over 20 h NaCl treatment. Ten-day-old seedlings were treated with (dotted line) or without (solid line) 100 mM NaCl at ZT0.TUBULIN2 (TUB2) was used as internal control. Data represent the mean±s.e. of three independent experiments. White-and-black bar represents light and dark periods, respectively. (e) Na+/H+exchange activity in plasma membrane vesicles isolated from WT,gi-1andsos1-1leaves is shown as a function of Na+concentration in the assay medium. Each point is the average of three technical replicates ±s.d. (f) SOS1 abundance increased in thegimutant. Leaves of 3-week-old WT, SOS1-OX,gi-1and SOS1-OX ×gi-1plants were treated with 100 mM NaCl for 24 h. SOS1 was detected in total protein extracts by immunoblotting with anti-SOS1 antibody. Molecular weight markers in kDa. The CBB-stained membrane is shown as a loading control. The bottom two panels represent RT–PCR analysis of theSOS1andTUBULIN2(TUB, control) transcript levels in these leaves. All experiments were repeated at least three times. Figure 2: Salt tolerance in the gi mutant is mediated by increased Na + /H + exchange activity. ( a , b ) The gi mutant exhibits increased salt tolerance. ( a ) WT, gi-1 and GI-OX plants were grown on soil for 3 weeks (top panel) and then treated with 0 mM (middle) or 150 mM (bottom) NaCl for 2 weeks. Plants are shown ( a ) representative of 10 to 12 individual plants that were examined for each line. ( b ) Fresh weight at the end of the treatments shown in ( a ). Index indicates the per cent decrease in average fresh weight after NaCl treatment. Data represent the mean±s.e. of the three independent replicates. ( c , d ) qRT–PCR analysis of P5CS1 ( c ) and DREB2A ( d ) transcript levels over 20 h NaCl treatment. Ten-day-old seedlings were treated with (dotted line) or without (solid line) 100 mM NaCl at ZT0. TUBULIN2 (TUB2 ) was used as internal control. Data represent the mean±s.e. of three independent experiments. White-and-black bar represents light and dark periods, respectively. ( e ) Na + /H + exchange activity in plasma membrane vesicles isolated from WT, gi-1 and sos1-1 leaves is shown as a function of Na + concentration in the assay medium. Each point is the average of three technical replicates ±s.d. ( f ) SOS1 abundance increased in the gi mutant. Leaves of 3-week-old WT, SOS1-OX, gi-1 and SOS1-OX × gi-1 plants were treated with 100 mM NaCl for 24 h. SOS1 was detected in total protein extracts by immunoblotting with anti-SOS1 antibody. Molecular weight markers in kDa. The CBB-stained membrane is shown as a loading control. The bottom two panels represent RT–PCR analysis of the SOS1 and TUBULIN2 ( TUB , control) transcript levels in these leaves. All experiments were repeated at least three times. Full size image Exposure of plants to stresses induces reprogramming of the transcriptome that reflects coping mechanisms. The P5CS1 gene and genes encoding transcription factors of the dehydration responsive element binding protein/C-repeat binding factor ( DREB/CBF ) family, such as DREB2A , are prominent among genes induced by numerous abiotic stresses and are considered as general stress response markers [3] , [30] . We considered the possibility that GI regulates a generalized stress response via transcriptional regulation. Comparison of the expression levels of P5CS1 and DREB2A in untreated and salt-treated WT, gi-1 and GI-OX plants by qRT–PCR analyses showed that salt stress-induced expression of these genes in all these lines, albeit with different kinetics and ZT maxima ( Fig. 2c ). In addition, we observed higher induction of DREB2A genes in gi-1 compared with WT, suggesting GI acts as a negative regulator of salt-induced DREB2A response even though the response of P5CS1 was not affected in the gi-1 mutant. P5CS1 and DREB2A transcript levels were dramatically changed in sos1-1 , as has been shown previously [31] ( Supplementary Fig. S8 ). Nonetheless, the induction of the DREB2A stress response gene was enhanced in gi-1 , this failed to explain the strong salt tolerance of gi-1 ( Fig. 2a ). Together with the fact that salinity controls GI at the posttranslational level ( Fig. 1d ), GI might affect the Arabidopsis growth response to salt by a mechanism involving transcriptional reprogramming of stress response genes and also through posttranslational control. Maintaining ion homeostasis under salt stress is another means for cells to survive. The plasma membrane Na + /H + antiporter SOS1 is a critical determinant of salt tolerance in Arabidopsis [31] . The Na + /H + exchanger activity of SOS1 is essential for Na + efflux from Arabidopsis cells. To ascertain whether GI affects SOS1 function, we measured the Na + /H + -exchange activity in purified plasma membrane vesicles from WT, gi-1 and sos1-1 plants. When compared with WT, Na + /H + -exchange activity was greatly reduced in vesicles of the salt-sensitive sos1-1 mutant, and was significantly higher in the salt-tolerant gi-1 mutant ( Fig. 2e ). Thus, GI appears to act as a negative regulator of salt tolerance by inhibiting Na + /H + exchanger activity of SOS1. To test whether SOS1 protein levels are affected by GI, we developed an anti-SOS1 antiserum that, albeit it was not completely SOS1 specific, it fails to recognize a protein corresponding to the predicted size of SOS1 (127 kDa) in extracts of sos1-1 plants ( Supplementary Fig. S4 ). This band is detected in WT and is more abundant in SOS1-OX plants. Using this antibody to estimate SOS1 protein levels, we observed that the gi-1 mutant accumulated SOS1 protein upon salt stress to a much higher level compared with WT without any evidence of an accompanying increase in SOS1 transcript level ( Fig. 2f ). The SOS1 overexpressing gi-1 (SOS1-OX gi-1 ) plants not only accumulated even higher amounts of SOS1 protein than gi-1 plants, but also exhibited more pronounced tolerance to salt than WT, SOS1-OX or gi-1 plants ( Figs 2f and 6a ). The salt tolerance of the gi-1 mutant compared with WT can thus be attributed to enhanced plasma membrane Na + /H + -exchange activity owing to the elevated level of SOS1 protein in the gi line ( Fig. 2e ). This conclusion is supported by studies in yeast mutants unable to excrete Na + that have clearly established the Na + /H + antiporter activity of SOS1 [7] , [9] , and by the observation that active SOS1 protein is a requirement for salt tolerance in Arabidopsis [32] . Figure 6: GI is involved in salt-sensitive signal transduction. ( a ) Seeds from indicated lines were grown on basal medium without (0 mM) or with 50 mM NaCl supplement under long-day conditions (16 h light/8 h dark) and photographed after 14 days. ( b – e ) Plants were grown on soil under the same long-day condition for 3 weeks (first row, before) and then (after) watered with water (0 mM NaCl) for 1 week (second row), 300 mM NaCl solution for 1 week (third row) or 300 mM NaCl solution for 2 weeks (fourth row). 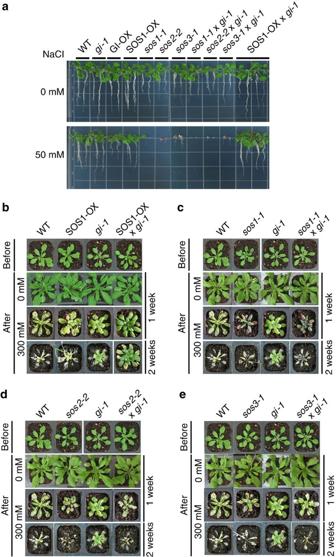Figure 6: GI is involved in salt-sensitive signal transduction. (a) Seeds from indicated lines were grown on basal medium without (0 mM) or with 50 mM NaCl supplement under long-day conditions (16 h light/8 h dark) and photographed after 14 days. (b–e) Plants were grown on soil under the same long-day condition for 3 weeks (first row, before) and then (after) watered with water (0 mM NaCl) for 1 week (second row), 300 mM NaCl solution for 1 week (third row) or 300 mM NaCl solution for 2 weeks (fourth row). Genotypes used: WT,gi-1, GI-OX (35S::GI-HA), SOS1-OX (35S::SOS1),sos1-1,sos2-2,sos3-1and double mutants SOS1-OX ×gi-1,sos1-1×gi-1,sos2-2×gi-1,sos3-1×gi-1. Genotypes used: WT, gi-1 , GI-OX ( 35S::GI-HA ), SOS1-OX ( 35S::SOS1 ), sos1-1 , sos2-2 , sos3-1 and double mutants SOS1-OX × gi-1 , sos1-1 × gi-1 , sos2-2 × gi-1 , sos3-1 × gi-1 . Full size image GI interacts with SOS2 GI is a partner in protein–protein interactions that affect functions of other proteins [25] , [33] , [34] . This led us to reason that GI may influence SOS1 function through direct or indirect protein interaction. To explore the interaction of GI with components of the SOS pathway in plants, we performed co-immunoprecipitation (co-IP) assays in leaf protein extracts from tobacco plants that were transiently expressing GI-HA with SOS1-GFP, SOS2-GFP or SOS3-myc fusions. The results showed that GI interacts with SOS2 and SOS3, possibly in a complex preformed in planta , whereas GI did not significantly interact with SOS1 ( Fig. 3a ). As SOS2 and SOS3 are known to interact in planta [8] , [9] , further tests determined whether one or both proteins interacted directly with GI. A pull-down assay using combinations of in vitro- translated 35 S-labelled GI protein and GST-SOS3, GST-SOS2 or GST (negative control) established that GI interacted strongly with SOS2 but not with SOS3 or GST ( Fig. 3b ). The interaction of GI with SOS2 but not SOS3 was confirmed using a yeast split-ubiquitin assay based on the reassembly of ubiquitin due to interaction of the fusion partners of its N- and C-terminal fragments (Nub and Cub). Only cells co-expressing Nub-SOS2 and GI-Cub-RUra3p were unable to grow on plates without uracil, but grew on plates containing 5-fluoroorotic acid (FOA), indicating that only SOS2 formed stable complexes with GI ( Fig. 3c ). 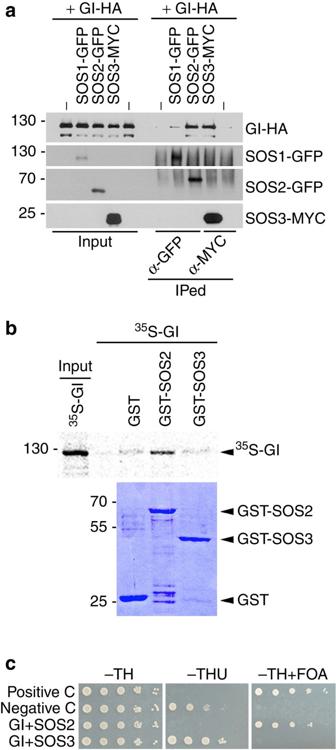Thus, GI interacts with SOS2 directly in vivo and in vitro . Figure 3: GI directly interacts with SOS2. (a) GI interacts with SOS2 and SOS3in vivo. Tobacco plants were infiltrated withAgrobacteriumharbouring35S::GI-HAand35S::SOS1-GFP,35S::SOS2-GFPor35S::SOS3-MYCfor transient expression. Protein extracts (Input) were immunoprecipitated (IPed) with anti-GFP or anti-MYC antibodies and resolved by SDS–PAGE. The shown immunoblots were developed with anti-HA to detect GI, anti-GFP to detect SOS1 or SOS2, and anti-MYC to detect SOS3 (b) GI interacts with SOS2in vitro. Shown is the autoradiograph (top panel inb) and CBB stain (bottom inb) of a gel containing resolved affinity-purified binding reactions that contained35S-GI, GST (negative control), GST-SOS2 and GST-SOS3 proteins in indicated combinations. Molecular weight markers in kDa. (c) GI interacts with SOS2 in the yeast split-ubiquitination assay. Positive and negative controls (c) represent yeast cells harbouring thepMet-SIZ1-Cub+pCup-NuI-SUMO1andpMet-Cub+pCup-NuIvectors, respectively. GI was fused to the N-terminus and either SOS2 or SOS3 were fused to the C-terminus of ubiquitin. Figure 3: GI directly interacts with SOS2. ( a ) GI interacts with SOS2 and SOS3 in vivo . Tobacco plants were infiltrated with Agrobacterium harbouring 35S::GI-HA and 35S::SOS1-GFP , 35S::SOS2-GFP or 35S::SOS3-MYC for transient expression. Protein extracts (Input) were immunoprecipitated (IPed) with anti-GFP or anti-MYC antibodies and resolved by SDS–PAGE. The shown immunoblots were developed with anti-HA to detect GI, anti-GFP to detect SOS1 or SOS2, and anti-MYC to detect SOS3 ( b ) GI interacts with SOS2 in vitro . Shown is the autoradiograph (top panel in b ) and CBB stain (bottom in b ) of a gel containing resolved affinity-purified binding reactions that contained 35 S-GI, GST (negative control), GST-SOS2 and GST-SOS3 proteins in indicated combinations. Molecular weight markers in kDa. ( c ) GI interacts with SOS2 in the yeast split-ubiquitination assay. Positive and negative controls ( c ) represent yeast cells harbouring the pMet-SIZ1-Cub + pCup-NuI-SUMO1 and pMet-Cub + pCup-NuI vectors, respectively. GI was fused to the N-terminus and either SOS2 or SOS3 were fused to the C-terminus of ubiquitin. Full size image This result suggested several possibilities for the function of GI as a negative regulator of salt tolerance. As the calcium-dependent SOS2–SOS3 protein complex activates SOS1, GI could either interfere with the SOS2-dependent upregulation of SOS1 or it could mask or disperse the influence of the sodium-sensing Ca 2+ -binding protein SOS3 (CBL4) on SOS2. It appeared also possible that the GI–SOS2 complex might have a specific function in the plant nucleus by which the transition to flowering is accelerated. In the latter, highly hypothetical scenario, GI would direct the normally cytosolically localized protein kinase SOS2 into the nucleus. GI inhibits SOS2-mediated SOS1 phosphorylation SOS2 encodes a serine/threonine protein kinase of the SNF1/AMPK family that activates the Na + /H + antiporter SOS1 through phosphorylation of SOS1 at its C-terminus (amino acids 441–1,146) [7] . To determine whether GI–SOS2 interaction affects phosphorylation of SOS1 by SOS2, an in vitro kinase assay was performed using a mutant SOS2 kinase (GST-SOS2 T168D ) [35] , [36] , which is more active than native SOS2 and is independent of SOS3. A C-terminal fragment of SOS1 was used as substrate. Inclusion of purified recombinant GI in the kinase reaction greatly reduced the phosphorylation level of SOS1, whereas the inclusion of BSA had no significant effect ( Fig. 4a ) leading to the conclusion that GI binds to SOS2 and renders it unavailable for SOS1 phosphorylation. The result was confirmed by demonstrating phosphorylation of SOS1 in vivo . SOS2-dependent phosphorylation of SOS1 in planta can be demonstrated in salt-stressed plants using anti-SOS1 antibody. Phosphorylated SOS1 is detected on immunoblots as a mobility-retarded band [7] . We detected significant amounts of the mobility-retarded, phosphorylated SOS1 band in the gi-1 and gi-201 plants compared with WT and SOS1-OX plants ( Fig. 4b ). 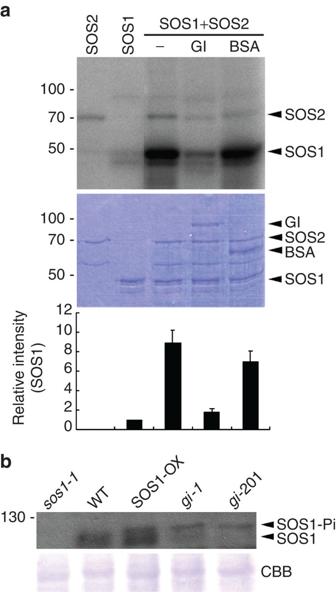Taken together, the in vitro and in vivo results revealed a negative effect of GI on SOS2-dependent phosphorylation of SOS1. Figure 4: GI inhibits SOS2-mediated SOS1 phosphorylation. (a) GI inhibits SOS2-mediated SOS1 phosphorylationin vitro.Anin vitrokinase assay was performed including purified bacterially expressed GST-SOS1 CD3 (SOS1 C-terminus, amino acids 885–1146), GST- SOS2T168D, MBP-GIN (GI N-terminus, amino acids, 1–391) and BSA (negative control) proteins in the indicated combinations. Shown are the autoradiogram (top panel) and CBB stain (middle) of a gel containing resolved reactions, and quantification of the SOS1 signals (n=3±s.d.; bottom panel). (b) Phosphorylated SOS1 protein accumulates in salt-stressedgiplants. Leaves of 3-week-old soil-grownsos1-1, WT, SOS1-OX,gi-1andgi-201plants were treated with 100 mM NaCl for 24 h. Immunoblot analysis of total protein extracts was performed with anti-SOS1 using CBB-stained bands as loading control. Molecular weight markers in kDa. Figure 4: GI inhibits SOS2-mediated SOS1 phosphorylation. ( a ) GI inhibits SOS2-mediated SOS1 phosphorylation in vitro. An in vitro kinase assay was performed including purified bacterially expressed GST-SOS1 CD3 (SOS1 C-terminus, amino acids 885–1146), GST- SOS2 T168D , MBP-GIN (GI N-terminus, amino acids, 1–391) and BSA (negative control) proteins in the indicated combinations. Shown are the autoradiogram (top panel) and CBB stain (middle) of a gel containing resolved reactions, and quantification of the SOS1 signals ( n =3±s.d. ; bottom panel). ( b ) Phosphorylated SOS1 protein accumulates in salt-stressed gi plants. Leaves of 3-week-old soil-grown sos1-1 , WT, SOS1-OX, gi-1 and gi-201 plants were treated with 100 mM NaCl for 24 h. Immunoblot analysis of total protein extracts was performed with anti-SOS1 using CBB-stained bands as loading control. Molecular weight markers in kDa. Full size image SOS1 phosporylation status is critical for SOS1 stability We next tested whether SOS1 stability was affected by its salt-induced phosphorylation status. A cell-free degradation assay was used consisting of the incubation of total protein extracts from salt-treated 35S::SOS1-HA plants with or without phosphatase. The relative degradation rate of HA-tagged SOS1 was measured by western blot analysis using anti-HA antibody. SOS1 protein levels declined more rapidly after phosphatase treatment indicating that the dephosphorylated SOS1 was more labile than its phosphorylated form ( Fig. 5a ). 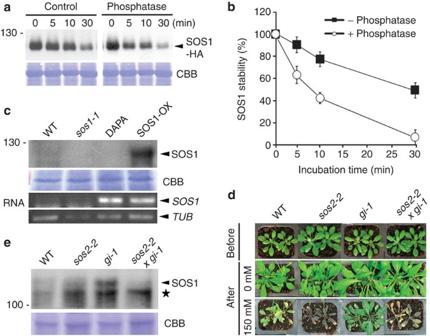This strongly suggested that salt stress-induced phosphorylation of SOS1 could have a role in stabilizing the protein. Figure 5: SOS2-dependent phosphorylation is critical for SOS1 protein stability and is increased in thegimutant. (a,b) Dephosphorylation of SOS1 increases its rate of degradation in cell extracts. Protein extracts of NaCl-treated (100 mM, 24 h) SOS1-HA-OX plants were incubated with lambda phosphatase at 30 °C for the indicated time periods in the presence (Control) or absence (Phosphatase) of phosphatase inhibitors and then subjected to immunoblot analysis with anti-HA antibody (upper panel). The CBB-stained bands are shown as loading control (lower panel). (b) Quantification of SOS1 protein levels shown in (a). Data represent mean±s.e. of three independent experiments. (c) SOS2-dependent phosphorylation is critical for SOS1 protein stability. Total protein extracts from NaCl-treated (100 mM, 24 h) leaves of 3-week-old WT,sos1-1, SOS1-OX-DAPA (overexpressing SOS1 mutated at the SOS2-target phosphorylation sites7) and SOS1-OX plants were subjected to immunoblot analysis with anti-SOS1 antibody. The CBB-stained bands provide a loading control. TheSOS1transcript level was confirmed by RT–PCR.TUBULIN2(TUB) transcripts (bottom row) provide a loading control. (d) SOS2 is required forgi-1-mediated salt tolerance. Shown are WT,sos2-2,gi-1, andsos2-2×gi-1double-mutant plants that were grown in long-day conditions (16 h light/8 h dark) on soil for 3 weeks (before) and then (after) watered with 0 mM (middle row) or 150 mM (bottom row) NaCl solution for 2 weeks. (e) SOS2 is necessary for accumulation of SOS1 ingi-1. Protein extracts ofsos2-2,gi-1, sos2-2×gi-1double mutant, and WT plants treated with 100 mM NaCl for 24 h were subjected to immunoblot analysis as in (c). (a,c,e) Molecular weight markers in kDa. Figure 5: SOS2-dependent phosphorylation is critical for SOS1 protein stability and is increased in the gi mutant. ( a , b ) Dephosphorylation of SOS1 increases its rate of degradation in cell extracts. Protein extracts of NaCl-treated (100 mM, 24 h) SOS1-HA-OX plants were incubated with lambda phosphatase at 30 °C for the indicated time periods in the presence (Control) or absence (Phosphatase) of phosphatase inhibitors and then subjected to immunoblot analysis with anti-HA antibody (upper panel). The CBB-stained bands are shown as loading control (lower panel). ( b ) Quantification of SOS1 protein levels shown in ( a ). Data represent mean±s.e. of three independent experiments. ( c ) SOS2-dependent phosphorylation is critical for SOS1 protein stability. Total protein extracts from NaCl-treated (100 mM, 24 h) leaves of 3-week-old WT, sos1-1 , SOS1-OX-DAPA (overexpressing SOS1 mutated at the SOS2-target phosphorylation sites [7] ) and SOS1-OX plants were subjected to immunoblot analysis with anti-SOS1 antibody. The CBB-stained bands provide a loading control. The SOS1 transcript level was confirmed by RT–PCR. TUBULIN2 ( TUB ) transcripts (bottom row) provide a loading control. ( d ) SOS2 is required for gi-1 -mediated salt tolerance. Shown are WT, sos2-2 , gi-1 , and sos2-2 × gi-1 double-mutant plants that were grown in long-day conditions (16 h light/8 h dark) on soil for 3 weeks (before) and then (after) watered with 0 mM (middle row) or 150 mM (bottom row) NaCl solution for 2 weeks. ( e ) SOS2 is necessary for accumulation of SOS1 in gi-1 . Protein extracts of sos2-2 , gi-1, sos2-2 × gi-1 double mutant, and WT plants treated with 100 mM NaCl for 24 h were subjected to immunoblot analysis as in ( c ). ( a , c , e ) Molecular weight markers in kDa. Full size image A functional SOS2 is required for phosphorylation of SOS1 upon salt stress [7] . Studies in Saccharomyces cerevisiae have established that two specific serine residues of SOS1, S1136 and S1138, are essential and sufficient for activation by SOS2 and re-establishment of cellular ion homeostasis [7] . The role of SOS2-dependent phosphorylation in SOS1 stabilization in vivo was therefore verified by comparing SOS1 protein levels in NaCl-treated leaves of WT, sos1-1 , SOS1-OX-DAPA ( 35S::SOS1 S1136A/S1138A ) and SOS1-OX plants. Indeed, NaCl-induced accumulation of SOS1 protein was observed in SOS1-OX but not in SOS1-OX-DAPA plants although the SOS1 transcript levels were comparable in these two lines ( Fig. 5c ). On the basis of this result, we hypothesized that GI prevents SOS1 phosphorylation by inhibiting SOS2 kinase activity. This predicates that the salt tolerance phenotype caused by the inactivation of GI should be SOS2 dependent. We generated the double mutant, sos2-2 gi-1 , and conducted tests for salt tolerance in soil with 5-week-old plants. Indeed, sos2-2 gi-1 double-mutant plants did not exhibit the salt tolerance of single gi mutants ( Figs 5d and 6a ). Similarly, gi -dependent salt tolerance was suppressed in the sos1-1 gi-1 and also in the null sos3-1 gi-1 mutant that is impaired in SOS2-dependent phosphorylation of SOS1 ( Fig. 6a ). The steady-state levels of SOS1 protein in the salt-stressed gi-1 mutant was higher than that in identically treated WT, sos2-2 and sos2-2 gi-1 plants, as expected if the effect of GI on the SOS1 level in planta is mediated via SOS2 ( Fig. 5e ). Thus, it appears that inhibition of the SOS2-dependent phosphorylation and stabilization of SOS1 is the basis of the negative regulatory role of GI in the SOS pathway. Salt and SOS3 affect the interaction between GI and SOS2 GI degrades as a result of salt treatment ( Fig. 1d ). To test whether its interaction partner, SOS2, is necessary for GI degradation, diurnal oscillation of GI level was examined in WT and sos2-2 plants expressing the GI::GI-HA transgene after treatment with 0 or 100 mM NaCl at ZT0 ( Supplementary Fig. S5 ). The GI::GI-HA plants express native level of HA-tagged GI [33] . In absence of salt, GI-HA protein oscillated strongly in both WT and sos2-2 , even though the overall level of GI was lower in sos2-2 than in WT. The fraction of GI degraded upon salt treatment was comparable in sos2-2 and WT. This suggests that SOS2 has no significant effect on salt-dependent GI degradation. We then investigated the effects of NaCl treatment on the steady-state level of the GI–SOS2 complex in vivo . Tobacco plants transiently expressing combinations of GI-HA and SOS2-GFP were treated or not with NaCl and protein extracts were subjected to co-IP analyses. Compared with untreated controls, the amount of GI found in the GI–SOS2 protein complex pulled down with anti-GFP antibody was significantly lower after NaCl treatment ( Fig. 7a ). Re-establishment of cellular ion homeostasis under salt stress is initiated by binding of the calcium sensor SOS3 to SOS2 (ref. 37 ) raising the possibility that SOS3 can compete with GI for binding to SOS2. co-IP assays performed as above revealed that the SOS2–GI interaction in planta was indeed abolished by overexpression of SOS3 ( Fig. 7a ). 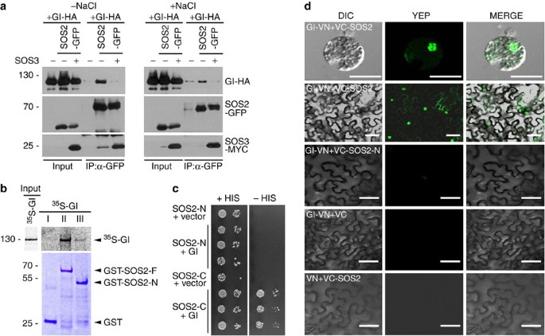Figure 7: Salt and SOS3 affect the interaction between GI and SOS2. (a) Salt and SOS3 interfere with GI–SOS2 interactionin vivo.35S::GI-HA, 35S::SOS2-GFPand35S::SOS3-MYCconstructs in the indicated combinations were transiently expressed in tobacco leaves byAgrobacteriuminfiltration. Shown are immunoblots of total protein extracts from leaves treated with 0 (−NaCl) or 100 mM NaCl (+NaCl) for 24 h that were fractionated by SDS–PAGE before (Input) or after immunoprecipitation with anti-GFP antibody (IP:α-GFP). Blots were developed using tag-specific antibodies. (b) GI interacts with the C-terminus of SOS2.In vitro-translated35S-GI was incubated with GST (I) or the fusion proteins GST-SOS2-F (II; full-length SOS2, 1–446 aa) or GST-SOS2-N (III; SOS2 N-terminal catalytic domain, 1–308 aa). After pull-down with glutathione-cellulose, the protein complexes were resolved by SDS–PAGE and detected by autoradiography and CBB staining. (a,b) Molecular weight markers in kDa. (c) GI interacts with the C-terminus of SOS2. Shown are the results of a yeast two-hybrid assay using full-length GI protein (GI) as prey and SOS2-N or SOS2-C (SOS2 C-terminal regulatory domain, 309–446 aa) as bait. Empty vector was used as a negative control prey. Decimal dilutions of three independent cultures co-transformed with GI and SOS2 constructs were plated. Growth without histidine supplementation (−HIS) indicates positive interaction. (d) GI interacts with the C-terminus of SOS2in vivo. Shown are the results of bimolecular fluorescence complementation (BiFC) analyses performed with constructs containing Venus fluorescent protein N-terminal (VN) alone or fused to GI (GI-VN) and constructs containing Venus fluorescent protein C-terminal (VC) alone or fused to SOS2-F (VC-SOS2) or SOS2-N (VC-SOS2-N). Shown are images of tobacco protoplasts (top row) and epidermal cell layers (rows 2–5) that were isolated from infiltrated leaves (Bars=50 μm). Figure 7: Salt and SOS3 affect the interaction between GI and SOS2. ( a ) Salt and SOS3 interfere with GI–SOS2 interaction in vivo . 35S::GI-HA, 35S::SOS2-GFP and 35S::SOS3-MYC constructs in the indicated combinations were transiently expressed in tobacco leaves by Agrobacterium infiltration. Shown are immunoblots of total protein extracts from leaves treated with 0 (−NaCl) or 100 mM NaCl (+NaCl) for 24 h that were fractionated by SDS–PAGE before (Input) or after immunoprecipitation with anti-GFP antibody (IP:α-GFP). Blots were developed using tag-specific antibodies. ( b ) GI interacts with the C-terminus of SOS2. In vitro -translated 35 S-GI was incubated with GST (I) or the fusion proteins GST-SOS2-F (II; full-length SOS2, 1–446 aa) or GST-SOS2-N (III; SOS2 N-terminal catalytic domain, 1–308 aa). After pull-down with glutathione-cellulose, the protein complexes were resolved by SDS–PAGE and detected by autoradiography and CBB staining. ( a , b ) Molecular weight markers in kDa. ( c ) GI interacts with the C-terminus of SOS2. Shown are the results of a yeast two-hybrid assay using full-length GI protein (GI) as prey and SOS2-N or SOS2-C (SOS2 C-terminal regulatory domain, 309–446 aa) as bait. Empty vector was used as a negative control prey. Decimal dilutions of three independent cultures co-transformed with GI and SOS2 constructs were plated. Growth without histidine supplementation (−HIS) indicates positive interaction. ( d ) GI interacts with the C-terminus of SOS2 in vivo . Shown are the results of bimolecular fluorescence complementation (BiFC) analyses performed with constructs containing Venus fluorescent protein N-terminal (VN) alone or fused to GI (GI-VN) and constructs containing Venus fluorescent protein C-terminal (VC) alone or fused to SOS2-F (VC-SOS2) or SOS2-N (VC-SOS2-N). Shown are images of tobacco protoplasts (top row) and epidermal cell layers (rows 2–5) that were isolated from infiltrated leaves (Bars=50 μm). Full size image SOS3 physically interacts with the protein kinase SOS2 via the SOS2 C-terminal regulatory domain that then abolishes auto-inhibition of phosphorylation of SOS2 (ref. 38 ). To test the nature of the competitive relationship between GI and SOS3, we examined whether this competition was centred on the SOS2 regulatory domain. Compared with full-length SOS2, the C-terminally truncated SOS2 protein (SOS2-N) showed reduced binding of GI in a pull-down assay with in vitro radiolabeled GI ( Fig. 7b ). Yeast two-hybrid experiments demonstrated that the C-terminal domain SOS2 (SOS2-C) interacts with GI ( Fig.7c ). Bimolecular fluorescence complementation experiments in tobacco confirmed that C-terminal truncation of SOS2 abolished SOS2–GI interaction and also demonstrated that specific interaction of GI with SOS2 occurs both in the cytosol and nucleus ( Fig. 7d ). The observation that SOS3 and GI bind to the same domain of SOS2 explains the competition between SOS3 and GI for interaction with SOS2. Here, we identify GI, originally described as a gene regulating flowering time, as a major component of the salt-stress adaptation pathway. The data fit into a model ( Fig. 8 ) of a novel, unexpected function for GI as a regulator of the salt stress response. This role of GI combined with its known role in flowering allows coordination of flowering time with the salinity stress status of the juvenile plant. According to the model, the crucial salinity defense module is the dynamic protein complex consisting of GI and SOS2 kinase, the activator of the Na + /H + antiporter SOS1. Although GI is predominantly nuclear localized, it is known to be constitutively present at low levels in the cytosol in all tissues [33] . Accordingly, the model ( Fig. 8 ) shows GI binding with SOS2 in the cytosol to inhibit the SOS2-dependent phosphorylation of SOS1. In the absence of salt stress, GI binds to and inhibits the SOS2 function, keeping the SOS system in a resting state. Upon salt stress, GI undergoes proteasomal degradation, releasing SOS2 for interaction with SOS3. This promotes generation of the SOS2–SOS3 complex that activates SOS1 to re-establish ion homeostasis [7] , [9] . A consequence of the NaCl stress-dependent degradation of GI protein is the frequently observed delay in the initiation of flowering, which connected both processes. The GI–SOS2 complex was also observed in the nucleus ( Fig. 7d ), but there is no evidence that the SOS pathway might control flowering time ( Supplementary Fig. S7 ). However, a role for the nuclear GI–SOS2 complex in controlling salt tolerance cannot be excluded. Hypothetically, this may explain the exceptional salt tolerance associated with the inactivation of gi . 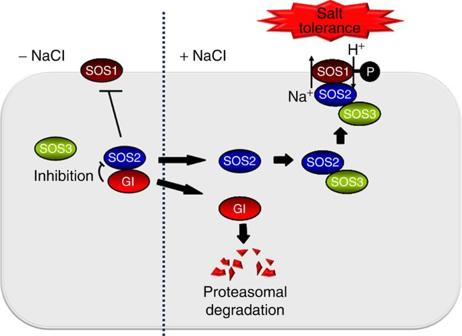Figure 8: A model for GI as a negative regulator of salt tolerance. In the absence of salt stress (−NaCl), GI binds to SOS2 and prevents interaction with the activating protein SOS3. Salt stress (+NaCl) triggers the degradation of GI, releasing SOS2. Free SOS2 then interacts with SOS3 to form an active SOS2–SOS3 protein kinase complex that translocates to the plasma membrane, allowing the SOS2-specific phosphorylation and activation of SOS1 that promotes salt-stress tolerance. Figure 8: A model for GI as a negative regulator of salt tolerance. In the absence of salt stress (−NaCl), GI binds to SOS2 and prevents interaction with the activating protein SOS3. Salt stress (+NaCl) triggers the degradation of GI, releasing SOS2. Free SOS2 then interacts with SOS3 to form an active SOS2–SOS3 protein kinase complex that translocates to the plasma membrane, allowing the SOS2-specific phosphorylation and activation of SOS1 that promotes salt-stress tolerance. Full size image GI has traditionally been associated with the promotion of flowering in long-day growth [24] , [25] , [27] , [28] . The genetic and biochemical mechanisms by which GI promotes flowering in long days are well-studied. GI was first identified in a screen for flowering time mutants in Arabidopsis . Since then deficiencies in GI have been shown to affect seedling photomorphogenesis in continuous red light [22] . gi lines affect the circadian clock and flowering time through controlling the stability of F-box proteins and transcription factor turnover. gi mutants show excessive starch accumulation, altered sucrose metabolism and enhanced sensitivity to light and oxidative stress [39] , [40] . Nonetheless, a molecular basis for the function of this protein has remained elusive as there are no known homologues outside plants, and there is no clear domain structure that might give clues to its function. Molecular interactors for GI, in the form of F-box proteins, have so far been identified in the context of the circadian clock and flowering. Another notable GI-interacting protein is SPINDLY, an O-linked N -acetylglucosamine transferase that negatively regulates flowering time and responses to growth-promoting GAs. SPINDLY appears to stabilize DELLA proteins, negative regulators of GA signalling, in an unknown way [41] , [42] . Arabidopsis plants lacking four DELLA genes are salt sensitive, whereas stabilized DELLA proteins enhance salt tolerance, but the precise connection between GI and DELLA-mediated salt tolerance, if any, remains unknown [4] , [5] , [6] . Our results, provide a clear molecular connection between the circadian clock, metabolism and salinity stress tolerance. In our model ( Fig. 8 ), GI conditionally interacts with the SOS2 protein kinase in the cytoplasm. This protein complex of conditional stability identifies the missing link between flowering and the specific adaptation to salt stress conditions. When our results are considered along with earlier reports [4] , [5] , [6] , [41] , [42] , it would appear that GI has a focal role from which other regulatory processes emerge to control vegetative growth rate, flowering time and stress tolerance. Through protein–protein interactions GI can be considered to act as a switch, partitioning and thus controlling diverse signalling intermediaries. Stability of GI would, in turn, determine the output of these pathways by sequestering or releasing interacting partners. The trigger that initiates flowering is connected to components of the circadian clock and regulated by the photoperiod to a large degree. Engrained circadian rhythmicity affects transcription of a large number of genes. In addition, multiple stress-response pathways are influenced by the circadian rhythm and flowering, with cold responses and vernalization constituting well-studied examples [13] , [43] , [44] . GI regulates circadian rhythms by mediating light input to the clock. Transcript levels of the salt-induced RD29A (COR78) gene are known to oscillate with a peak at ZT8-10 in basal media [45] , [46] . We show that the salt-induced expression of RD29A is in fact gated by the clock and that the clock affects RD29A gene expression ( Supplementary Fig. S6 ). Of the genes known to be under circadian control 68% encode stress-responsive functions [45] . Arguably, a possibly important function of the clock could be to anticipate and also integrate emerging stress conditions. The recognition of the interaction between vegetative growth, flowering and salinity tolerance provided here should influence strategies for the creation of salt-tolerant plants. The level of salt tolerance attained through the loss of GI is exceptional, exceeding the effect observed by the overexpression of SOS1 in Arabidopsis [47] . This could suggest that the role of GI in recruiting abiotic stress protection may extend beyond its effect on SOS2. Our results can be expected to initiate entirely new research directions in the understanding and manipulation of salt tolerance in crop plants. Plant materials and salt stress treatments A. thaliana mutants and transgenic lines sos1-1, sos2-2, sos3-1 , SOS1-OX, SOS1-HA-OX gi-1, gi-2, gi-201 , GI-HA-OX and GI::GI-HA were in Columbia ( Col-0 ) background [29] , [33] , [38] . Lines gi-1 sos1-1, gi-1 sos2-2, gi-1 sos3-1, gi-1 SOS1-OX and sos2-2 GI::GI-HA were generated by genetic crossing. Genotypes were verified by PCR and flowering times were recorded. Unless otherwise specified, plants were grown at 23 °C (16 h light per 8 h dark). To examine flowering time ( Fig. 1a ; Supplementary Figs S1 and S7 ), seeds were germinated and grown on basal medium (½ Murashige and Skoog (MS) salts, 2% sucrose) solidified with 1% agar, without or with NaCl supplement, in growth bottles (500 ml; 14 cm in height; five plants per bottle) with good air exchange. Flowering time was measured either by counting numbers of leaves (rosette+cauline) when bolted stems were ~1 cm long, or as days to bolting. For testing salt-tolerant phenotypes ( Figs 2a and 5d ), seeds were germinated in basal medium and 10-day-old seedlings were transferred to soil. Seventeen-day-old plants on soil were watered with indicated concentrations of NaCl twice per week for 2 weeks. For immunoblot analysis ( Figs 1d , 2f , 4b and 5c ), leaves detached from 3-week-old soil-grown plants were treated with NaCl at ZT1 (Zeitgeber Time 1) and harvested at times indicated in the legends. For salt treatment of seedlings, 2-week-old seedlings grown on filter paper (Advantec) in basal medium were treated with 100 mM NaCl at ZT0 by flooding the filter paper on salt solutions and harvested at times indicated ( Figs 2c, d and 6 ; Supplementary Figs S3 and S6 ). NaCl treatment was restricted to ZT0-ZT4 as plants were most responsive to stress during this interval, as established by measuring NaCl-induction of RD29A transcript levels ( Supplementary Fig. S6 ). RD29A has been characterized as a strongly salinity upregulated transcript [48] . Plasma membrane isolation and Na + /H + antiport assays Vesicles were isolated from 5-week-old plants by two-phase partitioning [49] . Na + /H + antiport activity was measured at 30 °C as Na + -induced dissipation of the pH gradient established by the activity of the plasma membrane H + -ATPase in inside-out plasma membrane vesicles isolated from leaves of WT, gi-1 and sos1-1 plants. Changes in pH during the assay were monitored as quenching of the pH-sensitive fluorescent probe 9-amino-6-chloro-2-methoxyacridine (ACMA) [50] . Assays (1 ml) contained 20 μg of plasma membrane protein, 1 μM ACMA, 50 mM 1,3-bis(tris(hydroxylmethyl) methylamino)propane (BTP)-HEPES (pH 7.5), 3 mM ATP-BTP (pH 7.5), 250 mM mannitol, 50 mM KNO 3 and 0.075% Brij58. Reactions were equilibrated in the dark with stirring for 5 min before beginning monitoring. Assays were initiated by the addition of 3 mM MgSO 4 . After reaching steady-state baseline fluorescence, Na + transport was initiated by adding NaCl. The initial rate of dissipation (ΔF min −1 ) was measured by changes in fluorescence during the first 10 s after addition of Na + . Reactions were terminated by adding 10 mM (final concentration) of (NH 4 ) 2 SO 4 to dissipate any remaining ΔpH and obtain the maximum fluorescence (Fmax). Fluorescence was recorded in a fluorescence spectrophotometer with a thermostated, stirred cell (Hitachi model FL-2500) at excitation and emission wavelengths of 415 and 485 nm, respectively. Activities are expressed in arbitrary units as the relative change in fluorescence (ΔF/Fmax) min −1 mg −1 membrane protein). RNA isolation and expression analysis Total RNA was extracted using RNeasy Plant Mini Kit (Qiagen) and treated with DNase (Sigma). First-strand cDNA was synthesized using the Thermoscript RT–PCR System (Invitrogen). PCR amplification used e-Taq DNA polymerase (Solgent). Gene-specific primers are listed in Supplementary Table S1 . RT–PCR conditions were as follows: 94 °C for 2 min, 25 (for GI ) or 30 (for SOS1 ) cycles of 94 °C for 30 s, 54 °C for 30 s and 72 °C for 1 min, followed by 72 °C for 5 min. Conditions for CO, FT, P5CS1 and DREB2A ) were 95 °C for 5 min, 45 cycles of 95 °C for 10 s and 60 °C for 30 s, followed by 95 °C for 10 s, 65 °C for 5 s and 95 °C for 5 s. Amplified products were detected using Power SYBR Green PCR master mix (Applied Biosystems) in a Bio-Rad C1000TM Thermal Cycler. The efficiency value of amplification for each primer set was checked by measuring the abundance of transcripts from cDNA dilutions according to the manufacture guide book (real-time PCR applications guide, Bio-Rad). Each data point shown is the average of two independent amplifications of the same RNA sample run in the same reaction plate. At least two independent RNA samples for each genotype and condition were used. Cloning For details see Supplementary Methods . Preparation of recombinant proteins For details see Supplementary Methods . In vitro binding assays 35 S-Met labelled GI protein was generated using in vitro transcription/translation (TNT Quick Coupled Transcription/Translation System, Promega). 35 S-Met labelled proteins were incubated with equal amounts of GST, GST-SOS2 proteins, or GST-SOS3 and glutathione-cellulose beads for 1 h at 4 °C in 100 μl of binding buffer (20 mM Tris–HCl, pH 7.5, 100 mM KCl, 50 mM NaCl, 0.5% NP-40, 10% glycerol, 5 μg ml −1 BSA, 1% Triton X-100, 1 mM PMSF, 5 μg ml −1 leupeptin, 5 μg ml −1 aprotinin, 1 μg ml −1 pepstatin, 5 μg ml −1 chymostatin, 5 μg ml −1 antipain, 50 μM MG132, 1 mM DTT and phosphatase inhibitors (1 mM each of NaF and Na 3 VO 4 ). Beads were washed and re-suspended in 15 μl of 2 × SDS sample buffer. Proteins released were separated by 10% SDS–PAGE, gels vacuum-dried and radiolabeled proteins detected by Cyclone (Perkin Elmer). Kinase assay Kinase reactions were set up essentially as described [51] , [52] . Combinations of purified bacterially expressed GST-SOS1 CD3 (substrate), GST-SOS2 T168D , MBP-GIN(1-391) and BSA were incubated with 0.6 μl of [γ- 32 P] ATP (6 μCi) in kinase buffer (20 mM Tris-HCl, pH 7.5, 10 mM MgCl 2 , 0.5 mM CaCl 2 , 2 mM DTT) at room temperature for 1 h followed by the addition of 6 × SDS loading buffer. Separated by 8% SDS–PAGE, protein gels were stained, de-stained and dried and radiolabelled proteins visualized using a Cyclone phosphor-imager (Perkin Elmer) [35] , [36] . Bimolecular fluorescence complementation assays Agrobacterium tumefaciens strain GV 3101 transformed with test constructs was grown in LB medium supplemented with 10 mM MES, 20 μM acetosyringone and antibiotics appropriate for particular constructs. Cells were collected by centrifugation and washed twice with infiltration solution (10 mM MgCl 2 , 10 mM MES and 100 μM acetosyringone). Agrobacterium cultures including cells harbouring p19 silencing plasmid was adjusted to OD 600 =0.5 in infiltration solution. Leaves of 4-week-old Nicotiana benthamiana plants were co-infiltrated with the desired combination of cultures and the plants were incubated for 2 days. Fluorescence of reconstituted YFP was detected using a confocal laser scanning microscope (Olympus FV1000) at excitation wavelength 515 nm. Immunoblot analysis and immunoprecipitation Protein was extracted in 100 mM Tris-Cl, pH 7.5, 150 mM NaCl, 0.5% NP-40, 1 mM EDTA, 3 mM DTT and protease inhibitors (1 mM PMSF, 5 μg ml −1 leupeptin, 1 μg ml −1 aprotinin, 1 μg ml −1 pepstatin, 5 μg ml −1 antipain, 5 μg ml −1 chymostatin, 2 mM Na 2 VO 3 , 2 mM NaF and 50 μM MG132) and separated on SDS–PAGE [33] . For analysis of SOS1 levels after phosphatase treatment, extracts were prepared either in 1 × phosphatase buffer supplemented with 2.5 mM MnCl 2 , 0.5% Triton X-100 and 0.4% Nonidet P-40, or in New England Biolabs (NEB) Buffer 3 with 5 μg ml −1 antipain, 5 μg ml −1 chymostatin, 1 μg ml −1 pepstatin, 5 μg ml −1 leupeptin, 5 μg ml −1 aprotinin, 1 mM PMSF, 50 μM MG132, 50 μM MG115 and 50 μM ALLN (acetyl- L -leucyl- L -leucyl- L -norleucinal). Aliquots (50 μl) of protein extracts were incubated with 400 units of lambda protein phosphatase (NEB) at 30 °C for 5 min in the absence or presence of phosphatase inhibitors (2 mM NaF, 2 mM Na 3 VO 4 ). Immunoblot analysis was carried out using rat α-HA (1:2,000; Roche) for SOS1-HA and GI-HA detection or mouse α-SOS1 (1:250) antibody. The antigen protein was detected by chemiluminescence using an ECL-detecting reagent (Thermo Scientific). Immunoprecipitation for interactions between GI and SOS proteins GI-HA and SOS1-GFP, SOS2-GFP or SOS3-MYC were transiently expressed in N. benthamiana leaf cells by Agrobacterium infiltration. For immunoprecipitation, rabbit anti-GFP polyclonal (1:250; Abcam) or mouse anti-MYC monoclonal (1:250; Cell Signalling Technology) antibodies were pre-incubated with protein A agarose (Invitrogen) at 4 °C. Then protein extracts (GI-HA and SOS1-GFP, GI-HA and SOS2-GFP, GI-HA and SOS3-MYC) were added and incubation continued for 1 h. Complexes were separated by SDS–PAGE and immunoblotted as described previously [33] . Each immunoblot was incubated with the appropriate primary antibody (anti-HA antibody, 1:2,000; anti-GFP antibody, 1:5,000; anti-MYC antibody, 1:1,000) for 4 h at room temperature or overnight at 4 °C. Membranes were developed using peroxidase-conjugated secondary antibody (1:1,000–3,000) (anti-rat IgG (Sigma), anti-mouse IgG (Santa Cruz Biotechnology), and anti-rabbit antibody (GE Healthcare)), and proteins were detected by ECL as described above. Yeast split-ubiquitin assay For split-ubiquitination assays [53] plasmids were transformed into S. cerevisiae strain JD53 using PEG and heat shock (Clontech protocol). Interactions between pairs of proteins were tested on selective medium containing 1.5 mg ml −1 5-FOA (5-Fluoroorotic acid monohydrate; Zymo Research) and selective medium lacking uracil. Plates were photographed after incubation at 30 °C for 3–5 days. Assays were each performed twice, and each experiment included three biological replicates. Interaction between GI and SOS2 For yeast two-hybrid assays, constructs were transformed into yeast strain HF7c. Growth of transformants was monitored on synthetic complete medium lacking Trp, Leu, +/− His. Three independent transformants of each SOS2 construct were tested for interaction with GI . Empty pACT2 provided the negative control. How to cite this article: Kim, W.-Y. et al . Release of SOS2 kinase from sequestration with GIGANTEA determines salt tolerance in Arabidopsis . Nat. Commun. 4:1352 doi: 10.1038/ncomms2357 (2013).